Stabilization of a linear nanomechanical oscillator to its thermodynamic limit The rapid development of micro- and nanomechanical oscillators in the past decade has led to the emergence of novel devices and sensors that are opening new frontiers in both applied and fundamental science. The potential of these devices is however affected by their increased sensitivity to external perturbations. Here we report a non-perturbative optomechanical stabilization technique and apply the method to stabilize a linear nanomechanical beam at its thermodynamic limit at room temperature. The reported ability to stabilize a nanomechanical oscillator to the thermodynamic limit can be extended to a variety of systems and increases the sensitivity range of nanomechanical sensors in both fundamental and applied studies. Thermal noise is well known to be an ubiquitous and fundamental limit for the sensitivity of micro- and nanomechanical oscillators [1] , [2] , [3] . This noise arises from the unavoidable coupling of the mechanical device to a thermal bath [4] , which is responsible for a motion with random amplitude and phase [5] . A number of precision measurements based on using nanomechanical resonators, such as gradient force [6] , [7] , mass [8] , [9] , [10] and charge [11] detection or time and frequency control [12] , consist of detecting linear changes induced by the measured system on the phase of the coherently driven nanomechanical sensor [1] , [13] . These applications are thus theoretically limited by the random phase fluctuations related to thermal motion. Decreasing the effect of thermal noise can be accomplished by increasing the relative contribution of the coherent drive [1] . However, the latter has to be kept below a certain threshold, above which the mechanical oscillator becomes nonlinear [3] , [14] : At this threshold—typically defined as the 1 dB compression point [3] —thermal noise constitutes an irreducible sensing limit for linear nanomechanical measurements in the classical regime ( k B T ≫ ħ Ω M , with k B being Boltzmann's constant, T being the temperature, ħ being the reduced Planck constant and Ω M being the mechanical resonance frequency). In practice, even when driven close to their nonlinear onset, nanomechanical resonators presently operate far away from the thermal limit [8] , [15] , [16] , [17] . Although several proposals have been made [18] , [19] and implemented [20] , [21] , [22] to decrease this excess phase noise, they are based on oscillators being driven into the nonlinear regime and require specific operating conditions, thus making the schemes difficult to adapt for a general class of resonators. Here we introduce an approach that generally applies to nanomechanical resonators in the linear regime. This approach employs an auxiliary mechanical mode as a frequency noise detector, whose output is used to stabilize the frequency of the fundamental out-of-plane mode of a nanomechanical beam. Its experimental implementation enables quasi-optimal linear operation at room temperature, with an almost perfect external phase noise cancellation, as demonstrated for the nanomechanical beam driven just below its nonlinear onset. Hence, our system operates close to its thermodynamic linear sensing limit, meaning that neither technical improvements (for example, in displacement detection) nor a change in the resonator driving strength can improve the effective frequency stability of the linear oscillator. Our scheme can be readily incorporated into a variety of other systems used for applications in sensing [7] , [8] , [9] , frequency control [12] , parametric processes [23] , [24] or fundamental studies [25] , [26] . Device and stabilization scheme Our system consists of an integrated hybrid optomechanical transducer described in ref. 27 . Briefly, it consists of a 90 μm × 700 nm × 100 nm low dissipation nanomechanical beam made of high-stress silicon nitride (Si 3 N 4 ) placed in the near-field of a whispering gallery mode confined in a disk-shaped microcavity ( cf. Fig. 1a ). Laser light is coupled in and out of the oscillator with a tapered fibre. Mechanical motion is read out using the optomechanical interaction by placing the laser frequency at mid-transmission of the optical mode, such that the phase fluctuations of light induced by the mechanical motion are directly transformed into amplitude fluctuations readily detected with a photodiode [28] , [29] . 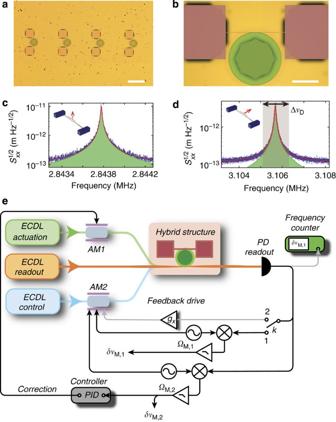Figure 1: The hybrid opto-nanomechanical system and experimental set-up. (a) Optical micrograph showing 4 of the 35 hybrid structures present on the chip used in the experiment (scale bar, 200 μm). (b) Magnified view of (a) showing the details of the hybrid structure (false colours; scale bar, 50 μm). (c) and (d) Thermal displacement spectraof the fundamental out-of-plane (mode 1) and in-plane (mode 2) modes, respectively. The green curves denote the thermal motion of the mechanical modes. The insets show finite-element simulations of the respective mechanical modes with the red arrows representing the direction of displacement. The grey area indrepresents the bandwidth ΔνDin which the stabilization scheme enables noise cancellation at the fundamental thermodynamical limit. In this bandwidth the detected thermal motion exceeds the contribution of the imprecision background. (e) Experimental set-up for the stabilization mechanism, with the readout and actuation of the mechanical oscillator being obtained via optical means with external cavity diode lasers (ECDL). The readout signal from the photodiode (PD) is split into a demodulation circuit for the directly driven noise detector mode 2 and a circuit for mode 1, which is either a directly driven (straight line) or self-driven (gray line) circuit. The self-drive of the oscillator is obtained by a feedback circuit (‘Feedback drive’), where the mechanical readout signal is phase-shifted by π/2, amplified and then applied as the excitation signal to the mechanics. Two amplitude modulators provide the means to drive the mechanical modes (AM2) and to control the mechanical frequency by changing the optical power coupled into the cavity (AM1). The frequency fluctuationsδνM,1andδνM,2are recorded either with an oscilloscope, when the system is operated in the direct driving mode orδνM,1is recorded with a frequency counter when the mode is self-driven. Figure 1: The hybrid opto-nanomechanical system and experimental set-up. ( a ) Optical micrograph showing 4 of the 35 hybrid structures present on the chip used in the experiment (scale bar, 200 μm). ( b ) Magnified view of ( a ) showing the details of the hybrid structure (false colours; scale bar, 50 μm). ( c ) and ( d ) Thermal displacement spectra of the fundamental out-of-plane (mode 1) and in-plane (mode 2) modes, respectively. The green curves denote the thermal motion of the mechanical modes. The insets show finite-element simulations of the respective mechanical modes with the red arrows representing the direction of displacement. The grey area in d represents the bandwidth Δ ν D in which the stabilization scheme enables noise cancellation at the fundamental thermodynamical limit. In this bandwidth the detected thermal motion exceeds the contribution of the imprecision background. ( e ) Experimental set-up for the stabilization mechanism, with the readout and actuation of the mechanical oscillator being obtained via optical means with external cavity diode lasers (ECDL). The readout signal from the photodiode (PD) is split into a demodulation circuit for the directly driven noise detector mode 2 and a circuit for mode 1, which is either a directly driven (straight line) or self-driven (gray line) circuit. The self-drive of the oscillator is obtained by a feedback circuit (‘Feedback drive’), where the mechanical readout signal is phase-shifted by π/2, amplified and then applied as the excitation signal to the mechanics. Two amplitude modulators provide the means to drive the mechanical modes (AM2) and to control the mechanical frequency by changing the optical power coupled into the cavity (AM1). The frequency fluctuations δν M,1 and δν M,2 are recorded either with an oscilloscope, when the system is operated in the direct driving mode or δν M,1 is recorded with a frequency counter when the mode is self-driven. Full size image Our stabilization scheme is based on the intuition that most of the observed external frequency noise in our system arises from perturbations affecting the entire beam geometry (for example, temperature fluctuations causing changes in length, strain among others). Under such conditions, the induced frequency fluctuations of the various eigenmodes are expected to be highly correlated. One of these modes can thus be used as a ‘noise detector’ whose output serves as an error signal in a feedback mechanism applied to the beam, enabling a cancellation of the geometry variations and thereby a stabilization of all eigenmodes ( cf. Fig. 2a ). A full quantitative description of the scheme is given in the Methods. In the following, our analysis will focus more specifically on two modes, which are the lowest-order out-of-plane mode, which we seek to stabilize, and the lowest-order in-plane mode, which is used as the noise detector. These two modes (referred to as mode 1 and 2, respectively, in the following) have resonance frequencies ν M,1 = Ω M,1 /2 π =2.84 MHz and ν M,2 = Ω M,2 /2 π =3.105 MHz as well as linewidths of Г M,1 /2 π =7.5 Hz and Г M,2 /2 π =48 Hz. Note that using the in-plane mode as the noise detector has several advantages: first, the accurate position resolution of the beam’s intrinsic motion enables to achieve a large bandwidth ( ν D ≃ 20 × Г M,2 /2 π ≃ 1 kHz, cf. Fig. 1d ) over which frequency fluctuations can be detected with thermal limited imprecision. Second, this geometry enables a selective exposure of the perpendicular out-of-plane mode to external signals, thus preserving its sensing capabilities when feedback is turned on. Experimentally, the frequency fluctuations of each mode are detected via its out-of-phase response to an external radiation pressure coherent drive with a frequency of Ω F, i ( i ε{1,2}), similar to a phase-locked-loop detection. The out-of-phase response corresponds to the dispersive response of the mechanical oscillator. We choose the driving strengths such that both modes have an amplitude of just below the respective nonlinear thresholds. Both measured out-of-phase quadratures for modes 1 and 2 are shown in Fig. 2d with the demodulated response plotted versus the detuning Ω i /2 π =( Ω F, i − Ω M, i )/2 π between the driving and the resonance frequency. By putting the external drive close to the resonance frequency ( Ω F, i ≃ Ω M, i ), we can monitor the resonance frequency as small changes on the order of δ Ω i ≲ Г M, i that are proportional to the out-of-phase quadrature signals. Our feedback mechanism relies on DC-photothermal actuation applied to the beam by sending a third, amplitude-modulated laser tone (control beam) with input power in the mW range (see Fig. 1e ). The frequency shift follows linearly the optical input power as shown in Fig. 2b for mode 1. 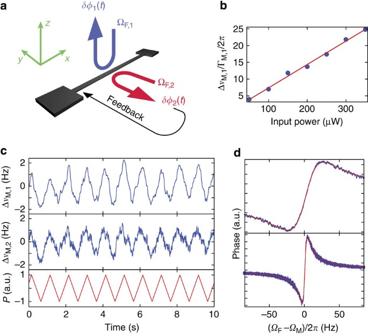Figure 2: Frequency stabilization with the optonanomechanical system. (a) Scheme describing the stabilization principle. Phase fluctuations of the in-plane mode (mode 2) are detected by determining its out-of-phase (dispersive) response to a coherent drive and serve as an error signal. By applying a feedback control based on these fluctuations, the out-of-plane mode (mode 1) is stabilized. (b) Resonance frequency shift ΔνM,1of mode 1 in terms of its mechanical linewidthΓM,1versus input optical power of the control field. (c) Resonance frequency shifts ΔνM,1and ΔνM,2of modes 1 and 2, respectively, for a saw-tooth modulation of the input optical powerPof the control field. The correlation of the response of both modes is clearly visible. (d) The out-of-phase mechanical response of mode 2 (upper graph) and mode 1 (lower graph) to a coherent drive versus the detuning (ΩF−ΩM)/2π. Figure 2: Frequency stabilization with the optonanomechanical system. ( a ) Scheme describing the stabilization principle. Phase fluctuations of the in-plane mode (mode 2) are detected by determining its out-of-phase (dispersive) response to a coherent drive and serve as an error signal. By applying a feedback control based on these fluctuations, the out-of-plane mode (mode 1) is stabilized. ( b ) Resonance frequency shift Δ ν M,1 of mode 1 in terms of its mechanical linewidth Γ M,1 versus input optical power of the control field. ( c ) Resonance frequency shifts Δ ν M,1 and Δ ν M,2 of modes 1 and 2, respectively, for a saw-tooth modulation of the input optical power P of the control field. The correlation of the response of both modes is clearly visible. ( d ) The out-of-phase mechanical response of mode 2 (upper graph) and mode 1 (lower graph) to a coherent drive versus the detuning ( Ω F − Ω M )/2 π . Full size image Figure 2c shows the frequency response of modes 1 and 2 to a triangular wave function applied to the control beam. One can already note the similarities of the fluctuations superimposed to the response triangles in both cases, indicating the common origin of the frequency noise over the various eigenmodes. These noise correlations can be quantitatively confirmed by determining the frequency correlations (with δν i [ Ω ] denoting the Fourier transform of the frequency fluctuations of mode i , its spectrum and ‹...› statistical average), which are represented in Fig. 3c (inset). It should be emphasized that in absence of external frequency noise, the frequency imprecisions caused by thermal noise over modes 1 and 2 are expected to be uncorrelated: the high level of correlations is therefore a signature of the presence of external frequency noise. 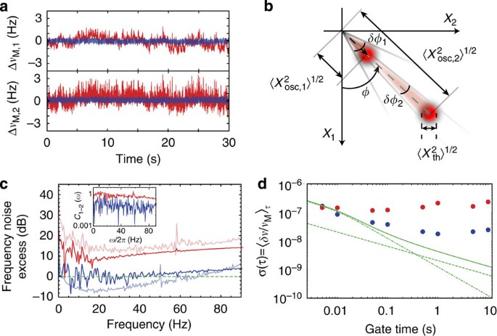Figure 3: Frequency stabilization at the thermodynamic limit. (a) Time evolution of the frequency driftδνMfor mode 1 (upper graph) and mode 2 (lower graph). The non-stabilized case is given by the red curve and the stabilized case by the grey one. (b) Thermal equivalent phase noise in phase space:X1andX2are the in-phase and out-of-phase components of mechanical motion, respectively, and form the phase space. In this representation, the phase of mechanical motion identifies to the azimuthal coordinateφ. The phase noiseδφsimply corresponds to the angle under which the thermal distribution appears from the centre. (c) Frequency noise excess of modes 1 (dark-coloured) and 2 (light-coloured) over the Fourier frequency components. The red and blue curves show the non-stabilized and stabilized case, respectively. The stabilization scheme reduces the frequency noise by over 10 dB up to 90 Hz and allows to stabilize mode 1 to the thermal limit for a wide bandwidth. Inset: The correlation of frequency response for both modes for the non-stabilized (red) and the stabilized (blue) case. (d) The fractional Allan deviation for the non-stabilized (red) and stabilized (blue) case. The dashed line shows the thermal limit associated with mode 1 for a self-driven oscillator. The dot-dashed line shows the thermal limit for mode 2, which was externally driven. The full line shows the thermal limit for mode 1 in presence of feedback (equation(4)) by taking into account the reinjected imprecision from mode 2. Experimentally, this excess of frequency noise is determined by comparing the phase noise spectrum S φφ,i [ Ω ] of mode i to its thermal equivalent imprecision, which in the strong drive limit is given by [2] , [5] Figure 3: Frequency stabilization at the thermodynamic limit. ( a ) Time evolution of the frequency drift δν M for mode 1 (upper graph) and mode 2 (lower graph). The non-stabilized case is given by the red curve and the stabilized case by the grey one. ( b ) Thermal equivalent phase noise in phase space: X 1 and X 2 are the in-phase and out-of-phase components of mechanical motion, respectively, and form the phase space. In this representation, the phase of mechanical motion identifies to the azimuthal coordinate φ . The phase noise δφ simply corresponds to the angle under which the thermal distribution appears from the centre. ( c ) Frequency noise excess of modes 1 (dark-coloured) and 2 (light-coloured) over the Fourier frequency components. The red and blue curves show the non-stabilized and stabilized case, respectively. The stabilization scheme reduces the frequency noise by over 10 dB up to 90 Hz and allows to stabilize mode 1 to the thermal limit for a wide bandwidth. Inset: The correlation of frequency response for both modes for the non-stabilized (red) and the stabilized (blue) case. ( d ) The fractional Allan deviation for the non-stabilized (red) and stabilized (blue) case. The dashed line shows the thermal limit associated with mode 1 for a self-driven oscillator. The dot-dashed line shows the thermal limit for mode 2, which was externally driven. The full line shows the thermal limit for mode 1 in presence of feedback (equation(4)) by taking into account the reinjected imprecision from mode 2. Full size image with being the variance of the driven amplitude, m eff, i being the effective mass, k B being Boltzmann’s constant, T being the temperature and Ω being the Fourier frequency. The phase noise spectrum is related to the frequency noise spectrum via S φφ [ Ω ]= S νν [ Ω ]/ ν 2 ( ν = Ω /2π). The detailed derivation of equation (1) is given in Supplementary Note 1 . Equation (1) simply reflects the fact that phase noise can be interpreted as the ‘angle’ under which the thermal distribution appears from the centre of the phase space (see Fig. 3b and Supplementary Fig. S1 ). Spectral analysis The time evolution of the frequency drift δν M, i , as determined from the mechanical out-of-phase response, is shown in Fig. 3a for mode 1 and mode 2. It is clearly evident that the frequency noise is strongly decreased for the stabilized case. These time traces are used to obtain the phase noise spectrum via a Fourier transform (details on calibration are given in Supplementary Note 2 ). In principle, the obtained spectrum corresponds to the determined phase noise versus the offset frequency from the mechanical resonance frequency. In order to visualize the excess noise, we have divided the data by the corresponding phase noise model given by equation 1. The results are shown in Fig. 3c , both in the non-stabilized (red) and stabilized (blue) cases. Dark coloured curves correspond to mode 1 and light coloured to mode 2. The results are calibrated using the inferred driven root-mean-square amplitudes =1.2 nm and =2.7 nm, just below their respective nonlinear thresholds (details of calibration are given in the Methods). When the system is not stabilized, the phase noise of both modes is clearly above the thermal limit. With the stabilization scheme turned on, the phase noise of mode 1 is reduced to the thermal limit in the frequency range of ~5–50 Hz. The spectrum of mode 2 implies that its phase noise was reduced to even below the thermal limit, which is clearly unphysical. This artefact arises from squashing, which is generally observed in an in-loop measurement when the feedback gain is so large that the reinjected background—in our case the thermally induced frequency fluctuations—is the dominating part of the error signal. A detailed model describing this effect is given in the Methods and its comparison to experimental data is shown in Supplementary Fig. S2 . As the spectrum of mode 1 is obtained in an out-of-loop measurement, reinjection of background would manifest itself correctly as an increase in the phase noise spectrum. As the thermal frequency noise background is smaller for mode 2 (28 mHz/ ) in comparison to mode 1 (41 mHz/ ), the reinjection of noise is limited for mode 1—the mode of interest—to a level of 1.5 dB with respect to the thermal limit. In these measurements, the readout noise [30] , [31] , [32] is negligible as described in detail in Supplementary Note 3 and shown in Supplementary Fig. S3 . We also observe the effect of stabilization on the correlations between the frequency noise of both modes. As noted above, noise suppression is expected to correspond to a significant decrease of the frequency noise correlations, as the noises resulting from fundamental thermodynamic fluctuations are uncorrelated. We confirm this experimentally as shown in the inset in Fig. 3c . Long-term stability To access the long-term stability for mode 1, we determine its Allan deviation. In order to avoid measurement artefacts, the mechanical motion is no longer driven using an external frequency reference, but is maintained in self-oscillation using a feedback circuit [27] , [33] (see Fig. 1e ). Briefly, a positive feedback is applied based on the measured mechanical signal, which is phase-shifted by π /2, amplified and then used as the excitation signal. The readout signal is fed into a frequency counter (A GILENT 53230), which determines the fractional Allan deviation as with as the averaged frequency in the k th discrete time interval over the gate time τ . The obtained results are shown in Fig. 3d , where the red and blue dots represent the values of the fractional Allan deviation of mode 1 as a function of gate time in the non-stabilized and stabilized cases, respectively. The slow fluctuations are significantly reduced in the presence of stabilization, with the noise suppression even exceeding 20 dB at the second scale. The achieved long-term stability is further compared with the theoretical limits of our system. For a self-sustained mechanical resonator, the thermo-mechanically limited Allan variance can be shown to be given by (see Supplementary Note 4 and Supplementary Fig. S4 ): The data of Fig. 3d were acquired in presence of a self-sustained displacement . This analysis shows that our stabilization scheme enables reducing external frequency noise close to the thermal limit, but not closer than a factor of 2 (that is, 6 dB in power), which disagrees with the spectral data of Fig. 3c . This can be explained by a reduced sensitivity of noise detection: Mode 2 being externally driven, the expression of its thermal limited Allan deviation differs from mode 1 and is described by (see Supplementary Note 4 ): With , the noise detection imprecision is comparable to (equation (2)), and therefore has to be taken into account when determining the stabilization limit, which is given by: The thermal limit for mode 2 as well as the overall stabilization limit given by equation (4) are represented in Fig. 3d , showing very good agreement with the experimental data up to gate times in the 100 ms range. On longer timescales, the frequency fluctuations are stabilized to a flat level in the 10 p.p.b. range, which we attribute to insufficient gain. Quadrature-based frequency noise detection Finally, we analyse the frequency stability and its improvement with the stabilization scheme by using a third independent method based on a recent proposal [34] . Briefly, this method is based on the simultaneous measurement of both in-phase and out-of-phase quadratures X 1 ( t ) and X 2 ( t ) of the coherently driven mechanical motion. These quadratures are used to reconstruct the complex motion trajectory u ( t )= X 1 ( t )+ iX 2 ( t ) whose moments ‹ u n › can be shown to be insensitive to thermal noise, enabling the extraction and quantitative study of external frequency noise. Thus, the presence of external frequency fluctuations δ Ω M ( t ) is revealed by an anomaly of the absolute value of the complex ratio r =‹ u 2 ›/‹ u › 2 , with | r | falling below unity by an amount proportional to the frequency noise power. Indeed, the quadratures of the coherently driven motion write as the sum of a steady and a fluctuating part X 1,2 ( t )=‹ X 1,2 ›+ δX 1,2 ( t ). A straight forward expansion gives ‹ u 2 ›=‹ u › 2 +‹( δX 1 ) 2 ›−‹( δX 2 ) 2 ›+2 i ‹ δX 1 δX 2 ›. With the thermal contribution to the quadrature fluctuations being uncorrelated and with identical variances, the previous expression becomes , with denoting the quadrature fluctuations due to the presence of external frequency noise. For a resonantly driven system, the in-phase quadrature X 1 is maximum, and , ‹ u 2 › is thus reduced to the quantity . At the mechanical resonance frequency, r gives a direct access to the frequency noise power, with no calibration being required. 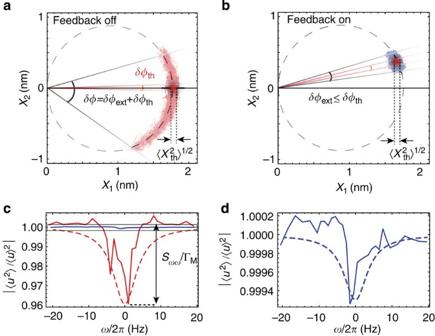Figure 4: Frequency noise self-characterization. (a) A realization of the phase-space trajectory acquired in the non-stabilized case when driving the nanomechanical beam at the mechanical resonance frequency (Ω≃0). The acquisition duration is 36 s. The red Gaussian disk represents the thermal distribution of variance, responsible for an equivalent phase noiseδφth.(b) Same as in (a), but for the stabilized case. The remaining phase noise clearly appears as being substantially reduced compared with non-stabilized case. (c) The ratio |‹u2›/‹u›2| for mode 1, which signifies the presence of frequency fluctuations due to non-thermal contributions, versus detuning from resonance frequency (red, nonstabilized; blue, stabilized). The red dashed line corresponds to the model given by equation (5) for a Gaussian noise with frequency power spectral density 15 dB above the thermal limit. Stabilization greatly reduces the dip due to excessive non-thermal noise. (d) Detailed view of |‹u2›/‹u›2| for the stabilized case. The blue dashed line corresponds to the model given by equation (5) for a Gaussian noise with power spectral density 1.5 dB above the thermal limit. In a more sophisticated approach [34] , it can be shown that for a weak Gaussian frequency noise with flat spectral density S Ω Ω , the ratio r [ Ω ] varies along the driving frequency as follows: Figure 4a,b shows the realizations of the phase-space trajectory used to determine r [ Ω ≃ 0] in the non-stabilized and stabilized configurations, respectively. Panels (c) and (d) show the experimental determination of r [ Ω ] we performed with our system, both in the non-stabilized ( Fig. 4c ) and in the stabilized cases ( Fig. 4c,d ). Figure 4: Frequency noise self-characterization. ( a ) A realization of the phase-space trajectory acquired in the non-stabilized case when driving the nanomechanical beam at the mechanical resonance frequency ( Ω ≃ 0). The acquisition duration is 36 s. The red Gaussian disk represents the thermal distribution of variance , responsible for an equivalent phase noise δφ th . ( b ) Same as in ( a ), but for the stabilized case. The remaining phase noise clearly appears as being substantially reduced compared with non-stabilized case. ( c ) The ratio |‹ u 2 ›/‹ u › 2 | for mode 1, which signifies the presence of frequency fluctuations due to non-thermal contributions, versus detuning from resonance frequency (red, nonstabilized; blue, stabilized). The red dashed line corresponds to the model given by equation (5) for a Gaussian noise with frequency power spectral density 15 dB above the thermal limit. Stabilization greatly reduces the dip due to excessive non-thermal noise. ( d ) Detailed view of |‹ u 2 ›/‹ u › 2 | for the stabilized case. The blue dashed line corresponds to the model given by equation (5) for a Gaussian noise with power spectral density 1.5 dB above the thermal limit. Full size image As expected, without stabilization we obtain a discernible dip around the mechanical resonance frequency as shown in Fig. 4c . The dip depth is about with the deviations from the expected shape resulting from long-term frequency drifts that change δ Ω . Following equation (5) such a dip is expected to correspond to a frequency noise , that is about 15 dB above the thermal limit , in very good agreement with the results presented in Fig. 3c . When the stabilization is switched on, the dip is greatly reduced to a level of , corresponding to a residual noise that is 1.5 dB above the expected thermal limit. This value confirms the origin of this remaining imprecision as resulting from squashing, which is expected to generate the very same noise excess as explained above. It is difficult to identify the exact origin of the excessive noise present in our system in its non-stabilized state. The excess of noise of 15 dB observed for the frequency noise spectra ( Fig. 3c ) and for the Allan deviation for a gate time of 1 s is already a good value for nanomechanical systems [8] , [15] . A possible reason is the integrated optical readout of mechanical motion, which allows to avoid noise resulting from the electrical readout [15] , [35] . We believe that the remaining noise is largely due to frequency shifts induced by random laser power fluctuations, which is reported to be a limiting factor in optically detected atomic force microscope cantilevers as well [36] . Frequency noise due to readout power fluctuations has also been recently reported in electrically readout nanoscale mechanical systems [37] . In conclusion, we have proposed and implemented a scheme allowing a non-perturbative stabilization of a mechanical mode. This technique proves to be remarkably efficient, as shown by the almost perfect noise cancellation for the lowest order out-of-plane mode of a high- Q nanomechanical resonator operated just below its nonlinear threshold, which places our system close to the optimum noise limit at room temperature. Our method is very general and can be readily applied to a number of ultra-sensitive nanomechanical systems: First, our scheme allows using any mechanical mode for detection of frequency noise and we successfully demonstrated noise cancellation using the third-order out-of-plane mode. To apply an error signal, one needs a DC restoring force, which is widely available either via photothermal forces in optomechanical systems such as in our work or as electrostatic forces in electrical systems [38] , [39] , [40] . Importantly, our scheme fully preserves the detection capabilities of the stabilized system. Theoretical description of stabilization scheme To theoretically describe the stabilization scheme, we consider the phase fluctuations δφ of the system, detected with the noise detector mode, against which we would like to stabilize. We can then write the stabilization feedback in frequency space as follows: where X th [ Ω ] denotes the mechanical thermal motion, δφ ext the phase fluctuations of the noise detector mode caused by external noise and g ν the stabilization feedback gain. The relationship for the phase fluctuations δφ given by equation (6) has three contributions given on the right-hand side of the equation. The first term describes the phase fluctuations resulting from the thermal motion of the mechanical oscillator, the second term describes the phase fluctuations resulting from external noise and the third term describes the stabilization feedback to counteract the phase fluctuations δφ . Here, the stabilization feedback response is low-pass filtered by the mechanical response function, with the filter width given by half of the mechanical linewidth of the noise detector mode. We can rewrite equation (6) as from which we can obtain the phase noise spectrum of the feedback stabilized mechanical mode to be where we have used the thermal displacement spectrum as given by equation (1) and where denotes the spectrum of the external phase fluctuations. We can describe the excess frequency noise as compared with the thermal limit by The last relationship given by equation (10) implies that in principle the stabilized phase noise spectrum can obtain values below the thermal limit, which—as noted previously—is clearly unphysical. This phenomenon can be explained by squashing, which is present for an in-loop measurement with high feedback gains and results from a reinjection of the readout background into the feedback loop. In the case described here, the readout background is given by the phase fluctuations resulting from thermal motion of the mechanical oscillator or, in other words, from the fundamental phase fluctuations. The above-derived relationships with the results given by equations (8) and (10) describe the decrease of phase noise in the noise detector mode corresponding to an in-loop measurement. However, we are in principle interested by the phase noise reduction of a different mode, namely the mode of interest. Assuming that the correlation of external frequency noise of both modes is close to unity, which holds true for our system, we can use the noise detector mode to reduce the phase noise of the mode of interest. We are now interested in the frequency fluctuations of the mode of interest, which, following the nomenclature introduced above, we denote by index 1, whereas the noise detector mode is denoted by index 2. As we use a different mode as the noise detector, the phase noise of the mode of interest is measured in an out-of-loop measurement, so that reinjection of background manifests itself correctly as an increase in the phase noise spectrum. With a calculation analogous to the in-loop case, we obtain which is valid for feedback gains well above one. This last relation shows that for high feedback gains g ν the reinjection of thermal noise from the noise detector mode adds up to the thermal noise of the mode of interest. It is thus of importance to keep the quantity as small as possible. Experimental validation of stabilization scheme Supplementary Figure S3 shows the excess of phase noise for modes 1 and 2 and corresponds in principle to Fig. 3b . The dark- and light-red curves refer to the non-stabilized modes 1 and 2, respectively. The blue curve refers to the stabilized mode 1 and the light blue curve to the stabilized mode 2. The green dashed curve denotes the thermal limit. As noted on the main text, we can observe a squashing artefact for the stabilized mode 2. We use our model described in equation (10) to obtain the expected squashing behaviour by taking the experimentally obtained data (light-red curve) for the ratio and values of Г M,2 /2 π =50 Hz and g ν ≃ 13.5 for the rest of the model, without any free parameter fitting. The result is plotted in black and shows an excellent agreement with the experimentally obtained squashed curve, thus validating both our model and our experimental results. Owing to squashing, we have in principle to take into account the reinjection of thermal background of mode 2 into mode 1 by the locking scheme, as described by equation (11). As we determine the thermal frequency noisse background to be smaller for mode 2 (28 mHz/ ) in comparison to mode 1 (41 mHz/ ), the reinjection of noise is limited for mode 1—the mode of interest–to a level of 1.5 dB with respect to the thermal limit. Stabilization of external actuation To demonstrate the efficiency of our stabilization scheme, we used it to counteract an externally applied actuation. The actuation corresponds to the one depicted in Fig. 2c and is derived from a saw-tooth modulation of the input optical power of the control field. As can be seen in Supplementary Fig. S5 , without stabilization the frequency response of the fundamental out-of-plane mode (mode 1) extends between −1.5 and 1.5 Hz (red curve). In case the stabilization is turned on, we can observe a drastic decrease of the frequency response to the actuation signal, which is still present. This is another demonstration of the efficiency of our stabilization scheme. Calibration and detection noise of mechanical motion We calibrate mechanical motion by detecting its displacement spectrum with an electronic spectrum analyzer (ESA). We calibrate the detected spectrum into absolute displacement using a phase-modulation technique [41] . From an evaluation of the detected spectrum, we can derive the amplitude of mechanical displacement as will be described below in more detail. We performed such a displacement calibration before each measurement of frequency noise with any of the three methods. For a thermally driven mechanical oscillator, the root-mean-square displacement is given by the well-known relationship [5] : For a practical system, T and Ω M can be determined in a straightforward manner. For the mass M , we need to assume an effective mass m eff [3] , [42] , which depends on the specific geometry of the mechanical system. For optomechanical near-field systems, such as the one used in our work, several studies [27] , [28] , [43] confirmed theoretically and experimentally that the effective mass corresponds to half of the physical mass. Thus, we can accurately determine the effective mass to be m eff ≃ 9 × 10 −15 kg. With T ≃ 300 K and Ω M /2 π ≃ 2.844 MHz, we obtain for the fundamental out-of-plane mode. To obtain the root-mean-displacement value of an externally driven mechanical mode, we compare the signal strength stored in the spectrum of this driven mode detected with an ESA with the corresponding signal strength stored in the thermal spectrum of this mode . As the bandwidth of the coherent source (Tektronix AFG3102) is much lower than the used resolution bandwidth of the ESA (1 Hz), the strength of the coherently driven signal is directly represented by its peak value . In case of the thermal motion, we need to integrate over the Lorentzian form of the oscillator and obtain a signal strength of . We can thus write with [Hz] denoting the units of Hertz. As we can determine by the calibration described above, we can obtain an absolute value for . However, for the most part only the ratio given by equation (13) is relevant, as can be seen from equations (1, 2, 3). In case the mechanical mode is self-driven via feedback, the ratio between the thermal and driven root-mean-square displacement is in principle given by [5] with Г eff as the effective linewidth of the self-driven mechanical oscillator [5] , [27] . In practice, for our implementation we use high feedback gains [5] , [15] , so that holds true and Г eff /2 π is once again well below the employed resolution bandwidth of the ESA (1 Hz) ( cf. Supplementary Fig. S6a ). Consequently, just as in the case with external driving, the signal strength of is confined to its peak value, so that we have to use once again equation (13) to determine the ratio between the thermal and driven root-mean-square displacements. We verified our hypothesis by fitting the resulting self-driven signal with a Gaussian function having a width of the ESA bandwidth and did indeed obtain a good agreement with the data as can be seen in ( cf. Supplementary Fig. S6b ). In contrast, fitting the data with a Lorentzian function, which is expected for a well-resolved self-driven signal, did not render an agreement. Detection noise of quadrature readout On the basis of a recent proposal [34] , we use the reconstruction u ( t )= X 1 ( t )+ iX 2 ( t ) of the in-phase and out-of-phase quadratures X 1 ( t ) and X 2 ( t ) to determine the excessive external noise present in our system. For each measurement point of Fig. 4c,d , we take a trace of 36 s. To estimate the readout uncertainty of mechanical motion, we first determine the readout dispersion Δ s th–th of the estimator s th–th (τ)=∫ 0 τ dt X th 2 ( t ) thermal motion ( τ is the averaging time) of a given quadrature using the relationship which was theoretically and experimentally established in ref. 27 and where the transfer function H res ( Г M , t ) is given by Using this relationship for our system parameters of τ ≃ 36 s and Г M /2 π ≃ 7.5 Hz, we determine a value of . This means that our readout imprecision of the thermally driven quadratures is about 5% of the root-mean-square value of thermal motion. In our experiments, we externally drive the mechanical motion with , so that the readout imprecision of the quadratures with respect to the detected driven motion is . As we use both quadratures to determine u ( t ), we can estimate the uncertainty of |‹ u 2 ›/‹ u › 2 | originating from thermal motion after an averaging time of 36 s to be on the level of 10 −6 of the measured value. The dip observed for the non-stabilized case ( Fig. 4c of main text, red curve) has a level of 4 × 10 −2 , which is well above the inferred imprecision. The dispersion of points in the non-stabilized case results from the frequency drifts of the mechanical resonance frequency Ω M /2 π and the corresponding detuning Ω /2 π between Ω M /2 π and the drive/demodulation frequency. This hypothesis is strongly corroborated by the significant reduction of dispersion for the stabilized case ( Fig. 4c of main text, black curve), as the stabilized mechanical resonance frequency leads to reduced fluctuations in Ω /2 π . In summary, we can conclude that readout imprecision does not have a role for this quadrature-based measurement of external noise. How to cite this article: Gavartin, E. et al. Stabilization of a linear nanomechanical oscillator to its thermodynamic limit. Nat. Commun. 4:2860 doi: 10.1038/ncomms3860 (2013).